Economic photoprotection in photosystem II that retains a complete light-harvesting system with slow energy traps The light-harvesting antenna of higher plant photosystem II has an intrinsic capability for self-defence against intense sunlight. The thermal dissipation of excess energy can be measured as the non-photochemical quenching of chlorophyll fluorescence. It has recently been proposed that the transition between the light-harvesting and self-defensive modes is associated with a reorganization of light-harvesting complexes. Here we show that despite structural changes, the photosystem II cross-section does not decrease. Our study reveals that the efficiency of energy trapping by the non-photochemical quencher(s) is lower than the efficiency of energy capture by the reaction centres. Consequently, the photoprotective mechanism works effectively for closed rather than open centres. This type of defence preserves the exceptional efficiency of electron transport in a broad range of light intensities, simultaneously ensuring high photosynthetic productivity and, under hazardous light conditions, sufficient photoprotection for both the reaction centre and the light-harvesting pigments of the antenna. Rational, artificial adjustment of the non-photochemical quenching (NPQ) process could improve the global crop yield by up to 30% (ref. 1 ), thus indicating the potential rewards associated with understanding the molecular mechanism(s) involved. The major protective, rapidly forming component of NPQ is called qE and depends on a light-induced ΔpH across the photosynthetic membrane, the de-epoxidation state of the xanthophyll cycle carotenoids and the presence of the PsbS protein in the membrane [2] . Modern qE theories commonly agree that structural changes within the photosynthetic membrane are behind the mechanics of the process. Initially, Bassi and colleagues [3] provided electron microscopy evidence that the distances between photosystem II (PSII) core complexes in detergent-solubilized grana membranes decreases under NPQ conditions. More recently, our group reported membrane reorganization occurring in intact chloroplasts exposed to high light, resulting in clustered domains of light-harvesting antenna (LHCII) and PSII reaction centres (RCII) [4] , [5] . Monomeric and trimeric antenna units, as well as the protein PsbS, were involved in the observed structural changes, which occurred on a timescale consistent with the formation and relaxation of qE. Following these electron microscopy-based observations, Holzwarth and colleagues [6] , [7] claimed that most of the LHCII complement of the membrane undergoes functional separation from the PSII core on formation of qE. This conclusion was based on the appearance of a red-shifted emission band in the decay-associated fluorescence spectra of illuminated leaves, absent in the dark, which was suggested to originate from quenched LHCII aggregates energetically separated from the PSII core [6] . Two NPQ quenching sites were proposed: one in the detached, aggregated cluster of LHCIIs, not in energy transfer contact with the RCs, the other in the remaining antenna complexes still attached to PSII [7] . Therefore, in light of this model PSII cross-section is expected to decrease during NPQ. However, it must be mentioned that a later work [8] on diluted chloroplasts did not reveal any long-wavelength components, which could be attributed to detached LHCII, although the resolution there was almost an order of magnitude higher than in the work of Holzwarth and colleagues [6] , [7] . Moreover, in the same work, low-temperature excitation fluorescence spectroscopy did not reveal any alterations in the PSII core antenna cross-section resulting from the detachment of chlorophyll b -enriched LHCII [8] . To explain the discrepancy, a few arguments can be raised on the validity of the methods used so far to assess the RCII cross-section. First, the conclusions by Holzwarth and colleagues [6] , [7] regarding a red-shifted emission component (due to detached LHCII) were not derived from a direct, genuine measurement of the fluorescence emission spectrum of LHCII in the NPQ state, but were based on a complex modelling of the time-resolved fluorescence of PSII and PSI, which required up to eight fluorescence lifetime components. Moreover, the lifetime measurements were performed on intact leaves. Under these conditions, a range of side effects occurs, which undermine the fluorescence data. One of them is photon re-absorption, known to distort the shape of the fluorescence spectrum and consequently to alter the decay-associated components [9] , [10] , [11] . Re-absorption by chlorophyll a dissolved in organic solvents at concentrations higher than 1 μM was shown to induce a distortion of the fluorescence lifetimes [12] . In a leaf, light scattering is also expected to increase absorption by the sample pigments, because it increases the optical path of light (detour effect), which in turn affects the fluorescence signal (for a review, see ref. 13 ). On the other hand, Holzwarth and colleagues [6] , [7] argued that the excitation fluorescence spectroscopy applied in ref. 8 was not a fit test of the RCII cross-section because of the strong overlap between PSII core and LHCII fluorescence, the measurements were performed at 77 K and the spectra were normalized at the chlorophyll a Soret band maximum. Taking into account all these controversial interpretations of the experimental observations, it seemed crucial to further investigate the important mechanistic point—whether the functional PSII antenna size changes during NPQ or not—with an independent approach. In the current study, using a millisecond fluorescence induction technique in the NPQ state compared with the dark-adapted state combined with the kinetic modelling of the photosynthetic membrane, we show that the functional antenna size of PSII during NPQ does not decrease. This brings the ‘strong-trap dogma’ and the existence of a pool of detached LHCII complexes, so far widely assumed for the NPQ mechanism, into question. Evaluation of PSII cross-section In the current work, the independent assessment of PSII cross-section in the NPQ state was based on two approaches. First, the antenna size was directly evaluated by applying Malkin’s method [14] (see below) to the fast fluorescence induction trace, measured from F o (open RCIIs) to F m (closed RCIIs) under weak light intensity and in the presence of 3-(3,4-dichlorophenyl)-1,1-dimethylurea (DCMU). This technique has been broadly applied in the past to determine static changes in PSII cross-section of different plant species (see for example ref. 15 ) but never for dynamically varying cross-sections. Next, to evaluate the PSII antenna size with a different approach, the fluorescence induction curve F ( t ) was fitted to a relevant mathematical model (for details see Supplementary Methods and Supplementary Fig. 1 ). According to the model, the photosynthetic membrane is made of heterogeneous PSII ‘puddle’ units [15] , hence F (t) is defined as follows: where, apart from photochemical excitation trapping by open and closed RCII (with the rates and , respectively), an additional channel of non-photochemical relaxation has been taken into account; k f is the fluorescence rate and P i ( j ) ( t ) is the probability that at a given time, i of N j RCIIs are closed. This model accounts for the possible heterogeneity of PSII antenna size [16] , as observed by freeze-fracture electron microscopy, ( Fig. 1c ), by summing over two variously-sized PSII subsystems, each having a weighting factor h j (see Supplementary Methods for more details). The fitting thus provides the following parameters for each fluorescence induction trace: p =1– k c / k 0 , which, in dark conditions, represents ( F m — F o )/ F m ; h j (the relative weight of each subsystem) and G j , the size of each subsystem, which, combined with h j , give the total cross-section G =∑ j h j G j . 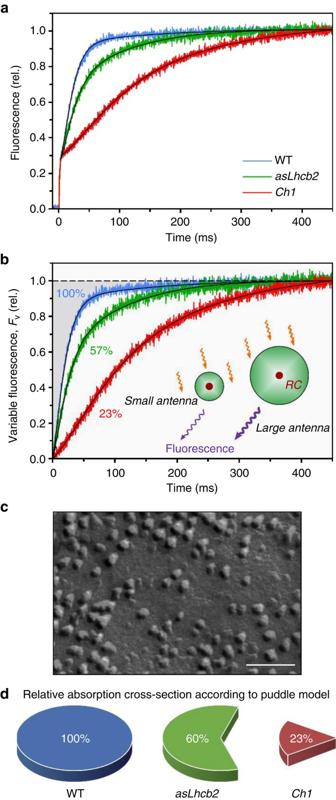Figure 1: Determining PSII cross-section inArabidopsismutants. (a) Representative fast PSII variable fluorescence induction traces of WT (blue),asLhcb2(green) andCh1(red)Arabidopsisleaves measured after infiltration with 30 μM DCMU and under 12 μmol photons per m2s−1. Model-based fittings are superimposed onto their respective traces (black lines). (b) The same traces as ina, but normalized to 1 atFmand zeroed atFo. The percentages correspond to the relative PSII cross-section size (1/(area above curve). (c) A freeze-fracture electron microscopy image of PSII-containing membranes showing the variations in RCII density as possible grounds for heterogeneity in PSII antenna size. Scale bar, 100 nm. (d) Pie charts showing relative differences between the mean absorption cross-sections in the WT,asLhcb2andCh1 Arabidopsisleaves, as obtained from modelling fluorescence induction curves. Figure 1: Determining PSII cross-section in Arabidopsis mutants. ( a ) Representative fast PSII variable fluorescence induction traces of WT (blue), asLhcb2 (green) and Ch1 (red) Arabidopsis leaves measured after infiltration with 30 μM DCMU and under 12 μmol photons per m 2 s −1 . Model-based fittings are superimposed onto their respective traces (black lines). ( b ) The same traces as in a , but normalized to 1 at F m and zeroed at F o . The percentages correspond to the relative PSII cross-section size (1/(area above curve). ( c ) A freeze-fracture electron microscopy image of PSII-containing membranes showing the variations in RCII density as possible grounds for heterogeneity in PSII antenna size. Scale bar, 100 nm. ( d ) Pie charts showing relative differences between the mean absorption cross-sections in the WT, asLhcb2 and Ch1 Arabidopsis leaves, as obtained from modelling fluorescence induction curves. Full size image Testing the validity of the method on PSII antenna mutants To illustrate the validity and consistency of the two approaches for the determination of the functional antenna size of PSII, wild-type (WT) Arabidopsis plants and two well-characterized mutants, antisense Lhcb2 ( asLhcb2) and Chlorina-1 ( Ch1) , have been used. The former mutant possesses a halved PSII antenna compared with the WT [17] , while Ch1 has no major LHCII and only expresses one monomeric antenna complex [18] . Taking into account that our WT plants formed ~5 LHCII trimers per one RCII [19] , it was possible to predict, on a biochemical basis [20] , [21] , that the chlorophyll content of the Ch1 antenna was ~22% that of the wild-type ( Table 1 , ‘Estimated cross-section’ column). Table 1 PSII cross-section in different types of Arabidopsis plants. Full size table Figure 1a shows the PSII fluorescence rise kinetics of DCMU-infiltrated leaves. Application of Malkin’s method to this data gives information on the size of the PSII antenna, which is in energy transfer contact with RCII, that is, the PSII cross-section, because the fluorescence rise time from F o to F m is inversely proportional to the antenna/RCII chlorophyll ratio. A change in the cross-section can be quantified, as described previously [14] , [22] , by directly calculating the area enclosed between the fluorescence induction curve ( F = F ( t )), the vertical axis ( t =0) and the maximal fluorescence level ( F = F m ), after normalizing the value of the variable fluorescence ( F v = F m — F o ) to unity ( Fig. 1b , the shaded area representing a relative value reciprocal to the RCII cross-section for a WT leaf). The asLhcb2 mutant showed slower kinetics than the WT, corresponding to a smaller cross-section (57% that of the control on average). The cross-section measured for the Ch1 leaf was only 23% that of the WT value, which is in good agreement with calculations based on biochemical data (see Table 1 ) and with a previous report [18] . According to our model-based results, the WT leaf consisted of two main pools of PSII, a large one (~400 chlorophylls per RC) besides a smaller pool of PSII supercomplexes, in agreement with the acknowledged existence of PSII centres with distinct photosynthetic unit sizes (the so-called α- and β-species of PSII [16] ). To fit the fluorescence induction traces of the mutants, it was necessary to increase the percentage of subsystems with smaller antenna size by ~27% for asLhcb2 and by ~37% for Ch1 (see black lines in Fig. 1a,b for obtained fits and Supplementary Table 1 for model parameters). A corresponding 40% and 77% decrease in total cross-section was found for asLhcb2 and Ch1 , respectively, in agreement with Malkin’s method and biochemical data ( Table 1 and Fig. 1d ). Assessing dynamic changes in PSII cross-section To verify the suitability of the method for monitoring a dynamically changing PSII cross-section, the induction of state transitions in WT leaves was employed. An alteration in environmental light quality causes an imbalance of energy input into PSI and PSII. State transitions work to correct this imbalance via a reduction of the size of the PSII antenna and a concomitant increase in PSI antenna size [23] , [24] , [25] , [26] . The phenomenon can be monitored using pulse amplitude modulation (PAM) fluorometry [27] . 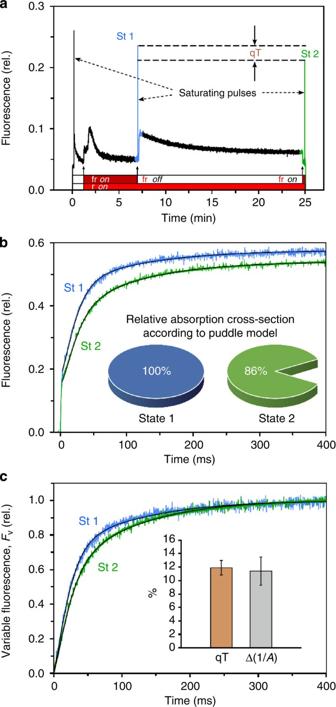Figure 2: Assessing state transitions as an example of dynamic changes of cross-section. (a) A typical state transition measurement of a spinach leaf performed via PAM fluorometry; ‘r’ and ‘fr’ denote red and far red lights, respectively. St 1 and 2 are states 1 and 2, respectively, reached as a result of red and far red light treatments, as indicated by on/off arrows and colour bars. First, St 1 was induced by illuminating the leaf with red (PSII) and far red (PSI) light of low intensity to avoid the formation of a proton gradient, NPQ and the saturation of the PSII reaction centres. After ~6 min, the far red light was switched off, causing a sharp rise in the fluorescence level due to overexcitation of PSII relative to PSI. The fluorescence started to decline and within ~15 min reached the steady-state level, St 2. At this point, part of the peripheral LHCII population becomes attached to PSI, thus increasing its cross-section and correcting the imbalance caused by the absence of far red light. (b) Fast PSII variable fluorescence induction traces measured in St 1 (in blue) and St 2 (in green) after infiltration with 30 μM DCMU and under 12 μmol photons per m2s−1. Model-based fittings are superimposed on to their respective traces (black lines). The pie charts illustrate relative differences between the mean absorption cross-sections in St 1 and St 2, as obtained from modelling fluorescence induction curves (seeSupplementary Table 2for the detailed model parameters). (c) Same traces as inb, but zeroed atFoand normalized to 1 atFm. The bar diagram shows the average amplitude of the state transition parameter qT, defined inaand obtained for the three independent measurements (brown bar), and decrease in PSII cross-section (Δ(1/A)) in St 2 relative to St 1 for three independent measurements (grey bar). Figure 2a shows a typical state transition trace. Leaves in states 1 and 2 were subject to measurements of fast fluorescence induction. The results are presented in Fig. 2b . A small, but still notable, decrease in the normalized fluorescence rise kinetics ( Fig. 2c ) can be seen for the leaf measured in state 2, consistent with the loss of RCII cross-section due to the migration of part of the peripheral antenna to PSI. Student’s test ( t -test) demonstrated that the difference between the two traces was statistically significant ( P =0.039). The decrease in the PSII cross-section was proportional to the decrease in F m ( Fig. 2c ), proving the validity of the method in detecting even small cross-section changes. The fitting-based model showed that on switching from state 1 to state 2, the weight of the subsystem with the smaller antenna size was increased by 8%, yielding a 16% reduction in PSII mean antenna size in state 2 compared with state 1 (see Supplementary Table 2 and Fig. 2b ), in good agreement with Malkin’s method. These results are quantitatively consistent with our actual knowledge of state transitions [23] , [24] , [25] , [26] . Figure 2: Assessing state transitions as an example of dynamic changes of cross-section. ( a ) A typical state transition measurement of a spinach leaf performed via PAM fluorometry; ‘r’ and ‘fr’ denote red and far red lights, respectively. St 1 and 2 are states 1 and 2, respectively, reached as a result of red and far red light treatments, as indicated by on/off arrows and colour bars. First, St 1 was induced by illuminating the leaf with red (PSII) and far red (PSI) light of low intensity to avoid the formation of a proton gradient, NPQ and the saturation of the PSII reaction centres. After ~6 min, the far red light was switched off, causing a sharp rise in the fluorescence level due to overexcitation of PSII relative to PSI. The fluorescence started to decline and within ~15 min reached the steady-state level, St 2. At this point, part of the peripheral LHCII population becomes attached to PSI, thus increasing its cross-section and correcting the imbalance caused by the absence of far red light. ( b ) Fast PSII variable fluorescence induction traces measured in St 1 (in blue) and St 2 (in green) after infiltration with 30 μM DCMU and under 12 μmol photons per m 2 s −1 . Model-based fittings are superimposed on to their respective traces (black lines). The pie charts illustrate relative differences between the mean absorption cross-sections in St 1 and St 2, as obtained from modelling fluorescence induction curves (see Supplementary Table 2 for the detailed model parameters). ( c ) Same traces as in b , but zeroed at F o and normalized to 1 at F m . The bar diagram shows the average amplitude of the state transition parameter qT, defined in a and obtained for the three independent measurements (brown bar), and decrease in PSII cross-section (Δ(1/ A )) in St 2 relative to St 1 for three independent measurements (grey bar). Full size image PSII cross-section increases during NPQ Measuring the fast fluorescence rise kinetics of PSII in the NPQ state is challenging due to the rapidity of qE relaxation. Vacuum infiltration of leaves with DCMU proved to be too slow to prevent NPQ recovery. A more suitable way consisted of the addition of DCMU directly into the incubation medium of intact, isolated chloroplasts (their intactness was assessed by light microscopy). The effective DCMU concentration yielding maximum F m was carefully determined by a titration of F m as a function of DCMU concentration (see Supplementary Fig. 2 and Supplementary Methods). Constant stirring ensured fast (within 5 s) delivery of DCMU in the sample cuvette ( Supplementary Fig. 3 and Supplementary Methods). A number of precautions were undertaken to ensure that NPQ relaxation did not occur during the assessment of the fluorescence induction trace. One of them was pretreatment of the leaves to induce up to 75–80% violaxanthin de-epoxidation. It was previously demonstrated that one of the factors, which can significantly slow down NPQ recovery, is the level of violaxanthin de-epoxidation or, equivalently, the concentration of zeaxanthin [28] , [29] . Accordingly, the time necessary for NPQ to relax in the presence of zeaxanthin is usually more than twice that in its absence ( Supplementary Fig. 3 ). As expected, enrichment in zeaxanthin caused in the dark adapted sample a decrease in the F v / F m ratio from 0.83 to ~0.7 (ref. 30 ) as well as a high level of NPQ, which took longer than 5 min to fully relax ( Fig. 3a ). The fast fluorescence induction measurement was therefore assessed within a time window where NPQ was high and constant (see magnified fluorescence induction part of the dark recovery on Fig. 3b showing the timing of fast fluorescence induction compared with the timing of NPQ relaxation). We proceeded as follows: after NPQ was induced for ~5 min, the actinic light and saturating pulses were turned off, DCMU was injected, the sample was continuously stirred in the darkness for 20 s to ensure complete action of DCMU (see Supplementary Fig. 3 ), then the low-intensity light that triggered the fast fluorescence rise in the NPQ state was applied (trace L, Fig. 4a ). In this way, an NPQ value (defined as ( F m — F m ′)/ F m ) of ~0.55 was found to be consistent in slow and fast kinetic mode (compare Fig. 3b with Fig. 4a , and also see Supplementary Fig. 4 where this comparison is made more explicitly). This result was interpreted as the fluorescence level measured in the NPQ state (L) being truly representative of F m ′. 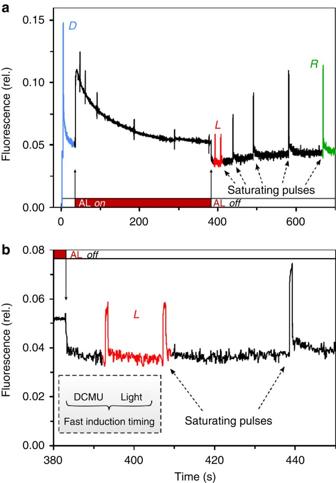Figure 3: Induction of a slowly relaxing NPQ. (a) A typical slow PAM fluorescence NPQ induction measurement performed on isolated intact spinach chloroplasts enriched in zeaxanthin. The actinic light intensity (AL) was 216 μmol photons per m2s−1. The different physiological states, where cross-section was measured, are marked withD(dark),L(NPQ state) andR(recovered, see alsoFig. 4). (b) The magnified region of dark recovery of the quenched fluorescence measured in the slow PAM fluorescence induction routine with indications of the timings of DCMU application and the illumination start in the fast fluorescence induction routine (‘light’) in the NPQ state (L). Saturating pulses having been used only in the slow induction routine to define the time window in which the levels of NPQ stayed constant during the fast fluorescence induction measurements. The insect shows that during the time window of cross-section assessment, NPQ level was constant. Figure 3: Induction of a slowly relaxing NPQ. ( a ) A typical slow PAM fluorescence NPQ induction measurement performed on isolated intact spinach chloroplasts enriched in zeaxanthin. The actinic light intensity (AL) was 216 μmol photons per m 2 s −1 . The different physiological states, where cross-section was measured, are marked with D (dark), L (NPQ state) and R (recovered, see also Fig. 4 ). ( b ) The magnified region of dark recovery of the quenched fluorescence measured in the slow PAM fluorescence induction routine with indications of the timings of DCMU application and the illumination start in the fast fluorescence induction routine (‘light’) in the NPQ state ( L ). Saturating pulses having been used only in the slow induction routine to define the time window in which the levels of NPQ stayed constant during the fast fluorescence induction measurements. The insect shows that during the time window of cross-section assessment, NPQ level was constant. 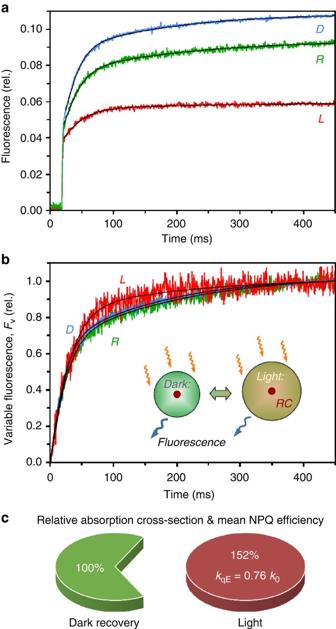Figure 4: Evaluation of PSII cross-section in NPQ state. (a) Fast PSII fluorescence induction traces performed on intact spinach chloroplasts following dark adaptation (D, in blue), illumination to induce NPQ (L, in red) and dark recovery of the fast NPQ component (R, in green) measured after addition of 6 μM DCMU and under 12 μmol photons per m2s−1. Model-based fittings are superimposed on to the respective traces (black lines). (b) Same as inaafter fluorescence traces were normalized to 1 atFmand zeroed atFo. (c) Pie charts showing relative differences between the mean absorption cross-sections for the light-adapted and dark-recovered intact spinach chloroplasts, and indicating mean NPQ efficiency in the light state, as obtained from modelling fluorescence induction curves. Full size image Figure 4: Evaluation of PSII cross-section in NPQ state. ( a ) Fast PSII fluorescence induction traces performed on intact spinach chloroplasts following dark adaptation ( D , in blue), illumination to induce NPQ ( L , in red) and dark recovery of the fast NPQ component ( R , in green) measured after addition of 6 μM DCMU and under 12 μmol photons per m 2 s −1 . Model-based fittings are superimposed on to the respective traces (black lines). ( b ) Same as in a after fluorescence traces were normalized to 1 at F m and zeroed at F o . ( c ) Pie charts showing relative differences between the mean absorption cross-sections for the light-adapted and dark-recovered intact spinach chloroplasts, and indicating mean NPQ efficiency in the light state, as obtained from modelling fluorescence induction curves. Full size image The fast fluorescence rise was also measured, for comparison, after qE was recovered in the dark ( R ) as well as for the dark-adapted chloroplasts before illumination ( D ). As a result, three sets of induction curves have been obtained with a representative set shown in Fig. 4a . Figure 4b shows F v rise traces for the three types of conditions, zeroed at F o and normalized to the maximum (as in Figs 1b and 2c ). Surprisingly, the fluorescence rise kinetics in the NPQ state was faster than in the dark, with an antenna size ~40% larger than in the dark state. We here point out that there was no sign of photoinhibition in the samples, as proven by the low fluorescence level after switching off the light (see Fig. 3 ). The increase in cross-section was therefore interpreted as a genuine consequence of NPQ induction in terms of structural changes within the membrane. As the light-induced increase in antenna size was a novel and somewhat unexpected result, the previously discussed modelling of fluorescence induction kinetics was applied to the ‘dark-recovered’ and ‘light’ states (see dark lines in Fig. 4a,b for fittings and Supplementary Table 3 for model parameters) for comparison. The theoretical model confirmed the increase in the antenna size in the NPQ state, being quantified as >30% larger than in the dark-recovered state (see Supplementary Methods , Supplementary Figs 5 and 6 , and Supplementary Tables 3 and 4 ), in close agreement with the results obtained from measured areas (Malkin’s method). Similar results were obtained for the dark state (before illumination) as expected from the similarity of the dark and recovered-dark traces of Fig. 4b . In this work we have reported on the assessment of PSII cross-section in the NPQ state. Direct measurements of the functional antenna size by Malkin’s method yielded results consistent with the model based on the fitting of the fluorescence induction traces. The two approaches have been validated by using a range of antenna mutants and, most importantly, for physiological dynamic antenna changes related to state transitions. We therefore concluded that an increase in the functional antenna size does occur during NPQ. This result disproves the hypothesis of energetic uncoupling of LHCII from RCII during NPQ as a consequence of the increased LHCII clustering [4] . It also contradicts the model [7] proposing functional detachment of up to 50% of the peripheral PSII antenna during NPQ, and fundamentally changes our collective understanding of the nature of the NPQ process. It has so far been assumed that to efficiently protect RCIIs, the exciton traps in the antenna must effectively ‘compete’ with excitation trapping by the RCII [31] . In this ‘strong trap’ scenario, the probability that an exciton reaches a RCII is significantly undermined by the appearance of traps within the antenna. As such strong traps should significantly reduce the functional size of the PSII antenna, one would expect the fluorescence induction in light to be notably slower than in the dark. However, our measurements indicate that this is not the case, and PSII antenna size is not reduced in the NPQ state. Although the total number of emitted photons was halved in the NPQ state (compare F m under light and dark conditions in Fig. 3a ), the kinetics of energy delivery from the antenna to the RCIIs was faster in light (in other words, it took less time for RCIIs to close). Moreover, our modelling directly indicates that in the PSIIs possessing the larger antenna, the NPQ is up to three times less efficient than the photochemical process, and the membrane-averaged NPQ trapping rate is ~75% of that of RCIIs (see Supplementary Table 3 ). As a result, the modelling allowed us to disentangle two terms related to the size of the light-harvesting antenna: the kinetic Malkin approach-based one (PSII cross-section) from what we call the efficiency of the antenna, representing the number of light-generated excitons used in RCIIs undermined by NPQ. This was quantified as follows. Under NPQ conditions, only k 0 /( k 0 +k qE )=(1+ Q ) −1 =57% of the light-generated excitation is trapped by open RCII. However, as the physical antenna size has increased by 52% ( Fig. 4d ), the efficiency of the antenna becomes 0.57 × 1.52=87% compared with the dark state. Thus, on switching to NPQ conditions, the efficiency of trapping by the open reaction centres decreased by only ~13%. Without such an adjustment of the antenna size, the drop in RCII efficiency would exceed 40%. At this point it is cogent to ask what all these findings tell us about the nature of the photoprotective response in PSII. First, they indicate the already mentioned increase in the energetically coupled PSII antenna following exposure to light; hence, rather than a functional disconnection of the peripheral antenna, we see that there is an increase in the overall connectivity of the membrane. Second, and more unexpectedly, our results revealed that the ‘strong trap’ picture of NPQ is not realistic, as the exciton traps that form within the PSII antenna appear to be rather inefficient, meaning that they hardly prevent energy from reaching open RCIIs. To understand how the presence of quenchers in the antenna affects the energy transfer dynamics of PSII, we must consider two limiting quenching regimes, the fast/slow (F/S) and the slow/fast (S/F) regimes. In the F/S regime, the transfer of energy from the antenna to the NPQ quenching site is fast (comparable to trapping by the reaction centres) but the dissipation of the trapped exciton is much slower (~100 ps). The chlorophyll–chlorophyll charge transfer state quenching model, for example, can be described as a F/S process [6] , [7] , [8] . In the S/F regime, energy delivery to the quencher is slow (~100 ps or even slower), while the dissipation of trapped energy is fast (~10 ps). The slow (20–30 ps) transfer of energy from Chla612 to lutein 620, leading to an effective trapping time of ~160 ps, followed by the rapid dissipation of the lutein S 1 excited state due to interconversion to the ground state is an example of the S/F regime [32] , [33] . The two regimes imply different extents of competition between photochemical and NPQ. In the F/S regime, trapping by the quenching sites competes effectively with the reaction centres. This competition would strongly undermine the amount of energy reaching the reaction centres. In the S/F regime, on the other hand, trapping by the quenchers is inefficient compared with open reaction centres and therefore does not prevent a significant amount of energy reaching the reaction centres before energetic equilibration in the antenna. Our results seem to support the S/F scenario. Nevertheless, the decrease in the total number of emitted photons in the NPQ state (see Fig. 4a ) demonstrates that the quenching is still effective on the timescale of PSII turnover (~10 ms). For these reasons, we suggest that the slow exciton traps in the antenna operate post factum , that is after antenna–RCII equilibrium is achieved. In summary, the fast F v rise kinetics represents a sensitive method capable of distinguishing between different processes occurring before and after energy equilibration in the antenna/RCII system. The fluorescence induction time from F o to F m can be viewed in terms of probability that photons hit the antenna before steady-state equilibration is reached: the bigger the antenna size, the higher the probability of photon absorption, the shorter the time taken to close all PSII reaction centres. Under NPQ conditions, this probability is higher, due to structural rearrangements, leading to a ~50% increase in the antenna size. Nevertheless, the total antenna efficiency is decreased by energy dissipation due to NPQ by only 13% (see above). This means that NPQ traps do not effectively prevent excitation energy reaching the reaction centres before their closure. Therefore, even in the quenched state, open reaction centres are still efficiently supplied with the excitation energy. The slow quenchers act only once energetic equilibration has been reached, serving to relieve the excitation pressure felt by the vulnerable closed reaction centres but not impeding the functionality of open ones. Slow traps capable of being generated everywhere in the antenna provide a flexible way to gradually adjust the overall efficiency of NPQ. We term this subtle mechanism economic photo-protection, as it is sufficient to protect the plant from photo-damage while not undermining the photosynthetic productivity. Plant material Arabidopsis thaliana cv Columbia WT, asLhcb2 (NASC ID: N6362) and Ch1 (NASC ID: N3119) plants were obtained from the European Arabidopsis Stock Centre. They were grown for 8–9 weeks in Sanyo plant growth cabinets with an 8-h photoperiod at a light intensity of 100 μmol photons per m 2 s −1 and a day/night temperature cycle of 22/15 °C. Chloroplast preparation Spinach was purchased from a local supermarket. Intact chloroplasts were prepared as previously described [34] , [35] . Chloroplasts devoid of zeaxanthin and antheraxanthin (V) were prepared from spinach leaves that had been dark-adapted for 1 h. To obtain a slowly relaxing NPQ, chloroplasts were enriched in zeaxanthin (Z) by pretreating leaves for 50 min at 350 μmol photons per m 2 s −1 under 98% N 2 /2% O 2 . Fluorescence induction measurements Chlorophyll fluorescence induction was measured with a Dual-PAM-100 fluorometer (Walz, Germany) on leaves and chloroplasts (17 μg ml −1 chlorophyll concentration) using the liquid cell adapter supplied with a cooling system at 18 °C. The chloroplasts reaction medium contained 0.3 M sorbitol, 20 mM tricine, 5 mM MgCl 2 , 2.5 mM EDTA pH 7.6. Methyl viologen (100 μM) was added as an exogenous electron acceptor after the first saturation pulse, before turning on the actinic light. Actinic illumination (216 μmol photons per m 2 s −1 ) was provided by arrays of 635 nm light-emitting diodes. The measuring light intensity was 12 μmol photons per m 2 s −1 . The maximum fluorescence ( F m ) was provided by a 0.8 s saturating light pulse (1,000 μmol photons per m 2 s −1 ). State transitions were measured in slow kinetics mode using 13 μmol photons per m 2 s −1 for the actinic light, 6 μmol photons per m 2 s −1 as measuring light and 76 μmol photons per m 2 s −1 far-red light (740 nm light-emitting diode). The fast fluorescence induction kinetic traces were measured with the same fluorometer using a custom-made trigger software (Waltz) providing a light flash of 12 μmol photons per m 2 s −11 intensity. For measures on leaves, dark-adapted samples were infiltrated with 30 μM DCMU, 150 mM sorbitol and 10 mM Hepes pH 7.5, immediately before running the fast kinetic programme. The effective DCMU concentration necessary to reach maximum F m was carefully determined for dark-adapted chloroplasts by measuring the fluorescence induction trace of samples containing gradually increasing DCMU concentrations (see Supplementary Fig. 2 ). The lowest concentration of DCMU at which the fluorescence level ceased to increase (6 μM) was considered to be saturating, and therefore used throughout the experiments. The kinetics of DCMU action was determined by using the method described in ref. 23 . Briefly, 6 μM DCMU was injected after ~5 min of illumination (216 μmol photons per m 2 s −1 ), then the time ranging from DCMU injection to the moment when fluorescence reached F m ’ was measured. This (~5 s, see also Supplementary Fig. 3 ) was considered as the time required for completing DCMU binding to PSII. For this reason, when measuring cross-section in the NPQ state, a gap of 20 s was fixed between DCMU injection and the fast fluorescence induction run (see also Supplementary Fig. 3 ). How to cite this article: Belgio, E. et al. Economic photoprotection in photosystem II that retains a complete light-harvesting system with slow energy traps. Nat. Commun. 5:4433 doi: 10.1038/ncomms5433 (2014).